Mid-range Ca2+signalling mediated by functional coupling between store-operated Ca2+entry and IP3-dependent Ca2+release The versatility and universality of Ca 2+ signals stem from the breadth of their spatial and temporal dynamics. Spatially, Ca 2+ signalling is well studied in the microdomain scale, close to a Ca 2+ channel, and at the whole-cell level. However, little is known about how local Ca 2+ signals are regulated to specifically activate spatially distant effectors without a global Ca 2+ rise. Here we show that an intricate coupling between the inositol 1,4,5 trisphosphate (IP 3 ) receptor, SERCA pump and store-operated Ca 2+ entry (SOCE) allows for efficient mid-range Ca 2+ signalling. Ca 2+ flowing through SOCE is taken up into the ER lumen by the SERCA pump, only to be re-released by IP 3 Rs to activate distal Ca 2+ -activated Cl − channels (CaCCs). This CaCC regulation contributes to setting the membrane potential of the cell. Hence functional coupling between SOCE, SERCA and IP 3 R limits local Ca 2+ diffusion and funnels Ca 2+ through the ER lumen to activate a spatially separate Ca 2+ effector. Calcium signalling is a ubiquitous signal transduction module that is operational in practically every cell type and species. Ca 2+ signals transmit information from various extracellular signals such as hormones, neurotransmitters and growth factors into defined cellular responses including cellular proliferation, fertilization and contraction [1] , [2] . Given the ubiquitous nature of Ca 2+ signals, the question arises of how a single messenger encodes such diverse cellular responses downstream of multiple agonists? Ca 2+ has unique features that allow it to specifically activate different cellular responses. Termination of the Ca 2+ signal involves either its removal from the signalling compartment—the cytosol— or buffering by mobile and immobile buffers. Specificity is encoded in the spatial, temporal, frequency and amplitude features of Ca 2+ transients, which are then translated into cellular responses by activating specific downstream Ca 2+ -dependent effectors [1] , [3] . Based on their spatial spread, intracellular Ca 2+ signals have been classified broadly as elementary (localized) or global [4] , with the latter referring to Ca 2+ signals that span the entire cell. Localized Ca 2+ signals are due to Ca 2+ flowing through Ca 2+ channels that creates a Ca 2+ microdomain with high Ca 2+ concentrations at the mouth of the channel, which gradually dissipates as Ca 2+ is buffered and is diluted as it diffuses into a larger volume [5] , [6] . The point-source Ca 2+ flowing through an open channel raises Ca 2+ to high levels, estimated to be on the order of 20–200 μM in the immediate vicinity of the channel, as Ca 2+ flow is too rapid to be captured by local Ca 2+ buffers [6] . Theoretical calculations argue that this point-source Ca 2+ rise decays rapidly in the spatial dimension due to Ca 2+ buffering resulting in a spatial spread estimated to be on the order of 20 nm (refs 7 , 8 ). In addition, Ca 2+ concentrations fall rapidly in the sub-micromolar range within 200 nm of the channel due to Ca 2+ buffering [7] , [9] , [10] . Experimental approaches have been developed to estimate the amplitude and spatial spread of microdomain Ca 2+ transients, including endogenous biological Ca 2+ sensors such as vesicle exocytosis and Ca 2+ -activated K + channels [11] , [12] , and optical single-channel imaging approaches using total internal reflection fluorescence (TIRF) and confocal microscopy [9] . In contrast to the Ca 2+ microdomain, global Ca 2+ signals work over larger distances of 10–100 μm. Both of these spatial ranges in Ca 2+ signalling have been investigated extensively, with presynaptic neurotransmitter release being the classical and best understood example of Ca 2+ action in the microdomain [7] . Several physiological examples argue that Ca 2+ signalling is effective in the mid-range between the local and global spatial extremes. Ca 2+ influx in lymphocytes controls the activation of transcription factors such as nuclear factor of activated T cells (NFAT), which do not localize in the Ca 2+ channel microdomain, with exquisite specificity [13] , [14] ; and Ca 2+ -activated K + channels are activated by Ca 2+ sources that are not in their immediate proximity [15] . However the mechanisms controlling mid-range Ca 2+ signalling, in the order of 0.5–5 μm, are not well defined. How does Ca 2+ flowing through localized channels activate spatially distal downstream effectors without inducing a global Ca 2+ rise? Ca 2+ diffusion alone will not be sufficient in this case given the high buffering capacity of the cytosol. It has been estimated that the effective range of free Ca 2+ ions in the cytosol is 0.1 μm before it is buffered [16] . As Ca 2+ levels rise from the resting levels of ~100 nM to the signalling levels of ≥1 μM, the diffusion coefficient of Ca 2+ increases fivefold, presumably due to saturation of the cytoplasmic buffering capacity [16] . Therefore, it is possible that mid-range Ca 2+ signalling can be achieved simply by modulating the flux through a channel (or channel cluster) to saturate local Ca 2+ buffers, and allow limited spread of the Ca 2+ signal. However, it is unclear how cells would be able to tightly control the Ca 2+ spatial spread, especially with the potential of Ca 2+ -induced Ca 2+ release through ryanodine and IP 3 receptors (IP 3 Rs) [17] . One well-defined mechanism in polarized pancreatic acinar cells is the so-called Ca 2+ tunnelling, where Ca 2+ entering through basolateral Ca 2+ channels flows through endoplasmic reticulum (ER) tunnels across the entire acinar cell to refill apical Ca 2+ stores [18] , [19] , [20] . Pancreatic acinar cells have a diameter of ≥15 μm, so it is difficult to think of Ca 2+ tunnelling as a mid-range Ca 2+ signalling module given the broad spatial extent it covers in a specialized polarized cell. Therefore, although it is clear that mid-range Ca 2+ signalling is functional in cells, the mechanisms underlying it remain obscure. To investigate potential mechanisms regulating mid-range Ca 2+ signalling, we studied the activation of Ca 2+ -activated Cl − channels (CaCCs) in Xenopus oocytes downstream of Ca 2+ influx. CaCCs are physiologically important for both the regulation of the oocyte membrane potential and the fast block to polyspermy at fertilization [21] . In addition to their well-established physiological roles in oocyte biology, CaCCs are important for many other cell physiological processes, including fluid secretion in epithelia and neuronal and cardiac excitability, and their biophysical properties have been well characterized in oocytes and other tissues [22] . Furthermore, the primary pathways controlling Ca 2+ dynamics in the oocyte are relatively simple compared with other cells and are well characterized [23] . Ca 2+ release from stores is mediated through the type 1 IP 3 R as the only ER Ca 2+ release channel expressed in the oocyte [24] . In addition, Ca 2+ influx occurs predominantly through store-operated Ca 2+ entry (SOCE) [25] , [26] , [27] following Ca 2+ store depletion. This leads to the clustering of STIM1, a Ca 2+ sensor enriched in the ER membrane with a lumenal EF-hand motif that senses Ca 2+ store content [28] , [29] . STIM1 clusters stabilize in a cortical ER domain just below the plasma membrane (PM) leading to the physical recruitment and gating of Orai1, a PM Ca 2+ channel [30] , [31] , [32] , [33] , [34] , [35] , [36] . Store refilling is mediated by SERCA pump, and Ca 2+ extrusion through the PM Ca 2+ -ATPase and potentially the Na + –Ca 2+ exchanger [37] , [38] , [39] . Hence, the relative simplicity of the Ca 2+ signalling machinery coupled to the existence of an endogenous physiologically important downstream Ca 2+ effector—the CaCC—makes the oocyte an attractive platform to investigate the regulation of mid-range Ca 2+ signalling. Here we show that functional coupling between SOCE at the PM and SERCA and IP 3 R at the ER membrane, efficiently directs focal Ca 2+ entry through SOCE channels to activate distant CaCCs. Differential activation of CaCC by Ca 2+ mobilizing agents CaCCs in the Xenopus oocyte provide an endogenous, sensitive and versatile reporter of Ca 2+ transients below the PM [40] . They faithfully report the temporal and amplitude changes in Ca 2+ dynamics as previously described [40] , [41] , [42] . Hence, CaCCs as endogenous physiological markers of Ca 2+ transients are superior to imaging approaches using Ca 2+ -sensitive dyes because they remove Ca 2+ buffering effects inherent to Ca 2+ dyes. Conveniently using a simple three-step voltage protocol CaCCs allow for the simultaneous monitoring of Ca 2+ release from stores through IP 3 Rs and Ca 2+ influx through SOCE ( Fig. 1a ) [25] , [40] . The first depolarizing pulse from a holding potential of −30 to +40 mV reports Ca 2+ released from stores as a sustained outward current termed I Cl1 ( Fig. 1a ). A second hyperpolarizing voltage jump to −140 mV drives Ca 2+ influx when SOCE is activated, triggering a time-dependent inward current termed I Cl2 ( Fig. 1a ). The third voltage jump to +40 mV results in a transient CaCC current termed I ClT , which is activated by Ca 2+ flowing through SOCE during the hyperpolarization pulse and gradually decays back to baseline ( Fig. 1a ). I ClT is calculated as the difference between I Cl1 and the maximal current measured during the second depolarizing voltage pulse ( Fig. 1a ), and has been shown to mirror sub-membrane Ca 2+ dynamics [40] . Importantly, these various currents are mediated by the same channel molecularly, TMEM16A or Anoctamin 1 (refs 42 , 43 ). 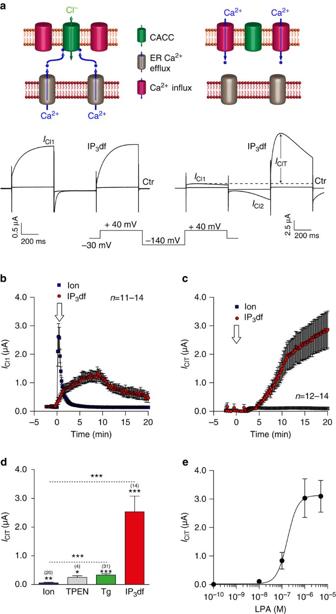Figure 1: Store depletion in the presence of IP3greatly enhances SOCE-dependent CaCC activation. (a) The sequential activation of CaCC in theXenopusoocyte allows the separation of Ca2+influx and Ca2+release. A triple-voltage jump protocol is used: the first pulse is a depolarization to +40 mV, allowing the recording ofICl1that reflects Ca2+release from intracellular stores (left traces and cartoon). The second pulse is a hyperpolarization to −140 mV, increasing the driving force for Ca2+influx. The third pulse is identical to the first one and measures the CaCC in response to Ca2+flowing during the preceding hyperpolarization pulse. (b) Injection of IP3df (final concentration ~100 nM) induces a slow transient intracellular Ca2+rise (grey circles), indicating the depletion of Ca2+stores. Ionomycin application (Ion, 10 μM, 20 s) induces a fast transient increase in intracellular Ca2+indicating rapid store depletion. (c)IClTdevelopment following store depletion with IP3df or ionomycin. (d) Summary ofIClTamplitudes following store depletion with different agents TPEN (5 mM, pre-incubated 30 min), thapsigargin (Tg; pre-incubated at 2 μM, 4 h in 50 μM Ca2+containing L15). (e) Bath application of lysophosphatidic acid (LPA) reproduces the effect of IP3df in a dose-dependent manner. Data are means±s.e.m., the number of cells tested is indicated next to the plots or above each bar. Statistics: *P<0.05, **P<0.01 and ***P<0.001; and NS, not significant. Figure 1: Store depletion in the presence of IP 3 greatly enhances SOCE-dependent CaCC activation. ( a ) The sequential activation of CaCC in the Xenopus oocyte allows the separation of Ca 2+ influx and Ca 2+ release. A triple-voltage jump protocol is used: the first pulse is a depolarization to +40 mV, allowing the recording of I Cl1 that reflects Ca 2+ release from intracellular stores (left traces and cartoon). The second pulse is a hyperpolarization to −140 mV, increasing the driving force for Ca 2+ influx. The third pulse is identical to the first one and measures the CaCC in response to Ca 2+ flowing during the preceding hyperpolarization pulse. ( b ) Injection of IP 3 df (final concentration ~100 nM) induces a slow transient intracellular Ca 2+ rise (grey circles), indicating the depletion of Ca 2+ stores. Ionomycin application (Ion, 10 μM, 20 s) induces a fast transient increase in intracellular Ca 2+ indicating rapid store depletion. ( c ) I ClT development following store depletion with IP 3 df or ionomycin. ( d ) Summary of I ClT amplitudes following store depletion with different agents TPEN (5 mM, pre-incubated 30 min), thapsigargin (Tg; pre-incubated at 2 μM, 4 h in 50 μM Ca 2+ containing L15). ( e ) Bath application of lysophosphatidic acid (LPA) reproduces the effect of IP 3 df in a dose-dependent manner. Data are means±s.e.m., the number of cells tested is indicated next to the plots or above each bar. Statistics: * P <0.05, ** P <0.01 and *** P <0.001; and NS, not significant. Full size image To test the effect of different Ca 2+ signalling modalities on the amplitude and kinetics of the CaCC current, we mobilized Ca 2+ stores and induced SOCE using various interventions. Mobilizing intracellular Ca 2+ using the non-hydrolyzable IP 3 analogue IP 3 df, induces a slow Ca 2+ release from stores as reported by I Cl1 ( t 1/2max =7.8±1.11 min, average±s.e.m., n =14) compared with the rapid release ( t 1/2max =0.58±0.15 min, n =11) observed in response to treatment with the Ca 2+ ionophore ionomycin ( Fig. 1b ). Although both Ca 2+ -mobilizing agents deplete intracellular Ca 2+ stores, the SOCE-dependent Cl − current ( I ClT ) is activated robustly only in response to IP 3 df but not ionomycin ( Fig. 1c,d ). Ionomycin induces a low-amplitude I ClT that was 30-fold smaller than that observed with IP 3 df ( Fig. 1d and Supplementary Fig. 1A,B ). Similarly to ionomycin, depleting stores through inhibition of SERCA pumps with thapsigargin results in a small I ClT as compared with the larger I ClT stimulated by IP 3 df ( Fig. 1d ). However, the thapsigargin-induced I ClT is ~4 times larger than that after ionomycin treatment (from 83.3±19 nA, n =20 for ionomycin to 329.5±48.4 nA, n =31 with thapsigargin; Fig. 1d ). These results argue that store depletion with IP 3 enhances the ability of CaCC to respond to Ca 2+ flowing into the cell through SOCE. To confirm that this effect is specific to IP 3 and SOCE, we activated SOCE with the low-affinity Ca 2+ chelator, TPEN, which is known to buffer free intraluminal ER Ca 2+ thus simulating store depletion [44] , [45] . In a similar manner to thapsigargin and ionomycin, TPEN failed to generate the large I ClT observed following IP 3 df treatment ( Fig. 1d ). Therefore, induction of large I ClT currents does not correlate with the extent or mode of store depletion but rather seems to require the presence of IP 3 . A potential explanation for the large amplitude of I ClT following injection of IP 3 df could be either the slow rate of Ca 2+ rise ( Fig. 1b ), or the Ca 2+ oscillations observed following this treatment. Conceivably, either of these Ca 2+ dynamics could activate signalling modules, such as kinases, leading to the differential modulation of I ClT . To test this possibility, we injected oocytes with high concentration of IP 3 (~2.5 μM), which results in rapid Ca 2+ release similar to what is observed with ionomycin, and leads to a large I ClT following store depletion ( Supplementary Fig. 1E ) [44] , [45] . We further treated cells with lysophosphatidic acid (LPA), which is known to activate G-protein coupled receptors and stimulate phospholipase C (PLC) to generate IP 3 in Xenopus oocytes [46] . The application of various concentrations of LPA (10 nM to 5 μM) releases Ca 2+ with different patterns, from a transient/oscillatory pattern for the lower concentrations to a large transient at higher concentrations ( Supplementary Fig. 1G–I ). The activation of I ClT by LPA was dose dependent and resulted, at high concentrations (1–10 μM), in I ClT amplitudes comparable to those recorded following IP 3 injection ( Fig. 1e ). These experiments indicate that the kinetics of Ca 2+ release do not significantly impact I ClT amplitude. The calcium release speed during application of 1 μM LPA ( t 1/2max =0.33±0.07 min, n =10), injection of IP 3 ( t 1/2max = 1.11±0.34 min, n =3) or ionomycin ( t 1/2max =0.58±0.15 min, n =11) are similar ( Supplementary Fig. 1 ), yet their ability to activate CaCC is markedly different. Ca 2+ oscillations generated by IP 3 df injection are also not required since the large single transient Ca 2+ release induced by IP 3 or 1 μM LPA is sufficient to trigger a large I ClT , similar to that observed with IP 3 df ( Supplementary Fig. 1D–F ). Taken together, these results suggest that in addition to SOCE, activation of the IP 3 R is critical for strong I ClT stimulation. SOCE amplitude is not affected by the store depletion mode As previously described, I ClT is activated downstream of SOCE [25] , [40] . Consistently, I ClT was inhibited by three pharmacological agents known to inhibit SOCE: Lanthanum, 2-APB (2-aminoethoxydiphenyl borate) and BTP-2 (3,5-bis(trifluoromethyl)pyrazole derivative) ( Supplementary Fig. 2 ). BTP-2 specifically inhibited I ClT without affecting I Cl1 showing that it does not affect Ca 2+ release from stores, and does not directly inhibit CaCC ( Supplementary Fig. 2E,F ). Given that I ClT is activated downstream of SOCE, the enhanced amplitude in response to IP 3 generation could be because of higher levels of SOCE. So we recorded the SOCE current ( I SOCE ) directly after store depletion with either ionomycin or IP 3 df ( Fig. 2 ). To record I SOCE , BAPTA was injected and effectively blocked the much larger I ClT ( Fig. 2a ). I SOCE was recorded using a voltage ramp as previously described [26] . Although the current showed a tendency towards higher amplitudes when induced by IP 3 df as compared with ionomycin, this was not significantly different ( Fig. 2b,c ), and as such could not account for the 30-fold increase in I ClT observed after IP 3 -dependent store depletion ( Fig. 1c ). Therefore, the enhanced activation of CaCC downstream of SOCE in cells where the IP 3 R is activated cannot be explained by enhanced SOCE amplitude. 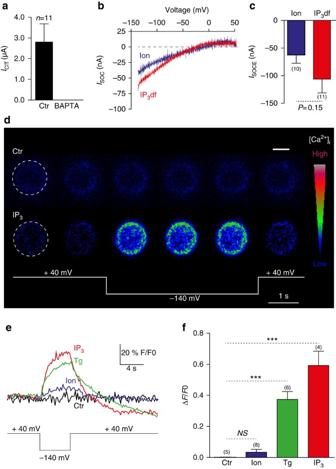Figure 2: SOCE current and cytoplasmic Ca2+in response to different Ca2+-mobilizing agents. (a) BAPTA (final 2.5–5 mM) was injected to uncouple intracellular Ca2+from CaCC resulting in a complete block ofIClT. (b) SOCE current–voltage relationship after store depletion with ionomycin or IP3df recorded in response to a voltage ramp from −140 to +50 mV as previously described26. (c) SOCE current amplitude (−140 mV) after store depletion with either ionomycin or IP3df. (d) To monitor intracellular Ca2+, oocyte loaded with Oregon green BAPTA-1 (40 μM) was injected with IP3, and simultaneous confocal imaging and voltage-clamp recording were performed. A voltage jump to −140 mV was used to maximize SOCE. An intracellular Ca2+increase during the hyperpolarizing pulse could be recorded in cells injected with IP3but not in control cells. Scale bar, 250 μm. (e) Time course of the intracellular Ca2+increase induced by a hyperpolarizing pulse to −140 mV when the intracellular stores were depleted with IP3, ionomycin (Ion) or thapsigargin (Tg). (f) Bar chart summarizing the Ca2+increase recorded as ine. Data are means±s.e.m., the number of cells tested is indicated above each bar. Statistics: ***P<0.001; and NS, not significant. Figure 2: SOCE current and cytoplasmic Ca 2+ in response to different Ca 2+ -mobilizing agents. ( a ) BAPTA (final 2.5–5 mM) was injected to uncouple intracellular Ca 2+ from CaCC resulting in a complete block of I ClT . ( b ) SOCE current–voltage relationship after store depletion with ionomycin or IP 3 df recorded in response to a voltage ramp from −140 to +50 mV as previously described [26] . ( c ) SOCE current amplitude (−140 mV) after store depletion with either ionomycin or IP 3 df. ( d ) To monitor intracellular Ca 2+ , oocyte loaded with Oregon green BAPTA-1 (40 μM) was injected with IP 3 , and simultaneous confocal imaging and voltage-clamp recording were performed. A voltage jump to −140 mV was used to maximize SOCE. An intracellular Ca 2+ increase during the hyperpolarizing pulse could be recorded in cells injected with IP 3 but not in control cells. Scale bar, 250 μm. ( e ) Time course of the intracellular Ca 2+ increase induced by a hyperpolarizing pulse to −140 mV when the intracellular stores were depleted with IP 3 , ionomycin (Ion) or thapsigargin (Tg). ( f ) Bar chart summarizing the Ca 2+ increase recorded as in e . Data are means±s.e.m., the number of cells tested is indicated above each bar. Statistics: *** P <0.001; and NS, not significant. Full size image Another formal possibility is that the CaCC Ca 2+ sensitivity is differentially regulated in response to distinct store depletion approaches, resulting in a better response to Ca 2+ entering through SOCE when stores are depleted using IP 3 . To directly activate the CaCC independently of other signalling modules, we injected Ca 2+ directly into the oocyte. As expected, Ca 2+ injection (70 pmol) activated I Cl1 , and importantly when Ca 2+ stores were depleted using ionomycin or IP 3 df no increase in I Cl1 could be observed, there was in contrast a significant reduction in I Cl1 after injection of IP 3 df ( Supplementary Fig. 3A,B ). Consequently, the increase in I ClT observed downstream of SOCE when IP 3 Rs are active cannot be attributed to an increased sensitivity of CaCC to Ca 2+ . Since CaCCs are activated by Ca 2+ below the cell membrane, the increased I ClT observed when IP 3 Rs are activated argues that a higher concentration of Ca 2+ is maintained in the sub-plasmalemal space leading to increased activation of CaCCs. So we directly visualized Ca 2+ dynamics downstream of SOCE activation in response to different Ca 2+ mobilizing agents, while simultaneously voltage clamping the cell ( Fig. 2d ). Hyperpolarization induced a larger Ca 2+ signal in IP 3 -injected cells as compared with cells treated with ionomycin ( Fig. 2d–f ). This reflects the recorded I ClT amplitude following IP 3 and ionomycin treatments ( Fig. 1d ). Hence I SOCE is similar when Ca 2+ stores are depleted with ionomycin or IP 3 , showing that the amount of Ca 2+ ions flowing into the cell in both cases is equivalent, yet IP 3 produces a larger cortical cytoplasmic Ca 2+ signal. This is likely due to Ca 2+ uptake into the ER by the SERCA pump in the case of ionomycin, thus preventing Ca 2+ accumulation in the cell cortex. To test this interpretation, we inhibited the SERCA pump with thapsigargin that resulted in Ca 2+ accumulation in the cytosol to significantly higher levels than with ionomycin and to equivalent levels to IP 3 ( Fig. 2e,f ). However, thapsigargin is ineffective at activating CaCCs to similar levels to IP 3 ( Fig. 1d ). These conflicting results argue that when IP 3 Rs are active, they act as a conduit to target Ca 2+ specifically to activate CaCCs. In the absence of IP 3 , Ca 2+ flowing through SOCE—as in the case of ionomycin-dependent store depletion—is taken up into the stores and does not significantly affect cortical cytoplasmic Ca 2+ levels ( Fig. 2d–f ), which would explain the low I ClT amplitude. Collectively, these results argue that functional IP 3 Rs are required for SOCE to activate CaCCs with high efficiency. To further test this conclusion, we depleted Ca 2+ stores with IP 3 df to maintain cytoplasmic IP 3 levels high. This results in store depletion as reported by I Cl1 , followed by the activation of SOCE and I ClT ( Fig. 3a ). After I ClT was fully activated, cells were injected with heparin to inhibit the IP 3 R ( Fig. 3a ). This results in complete inhibition of I ClT ( Fig. 3a ), showing that Ca 2+ release through IP 3 Rs is required for CaCC activation downstream of SOCE. These results argue that Ca 2+ flowing through SOCE is taken up into ER stores and then released again through IP 3 Rs to directly activate CaCCs. 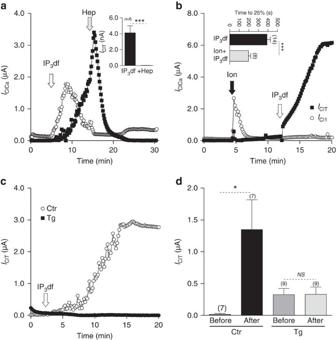Figure 3:IClTstimulation by IP3requires SERCA and active IP3R. (a) The injection of heparin (final concentration ~0.4 mg ml−1) inhibits theICITinduced by IP3df injection. (b) The injection of IP3df still potentiatesIClTwhen the stores have been previously depleted with ionomycin (ion). The inset shows a bar chart summary of the time required to reach 25% maximalIClTin control and ionomycin-pretreated cells. The data show a significantly more rapid rise (P<0.001) with ionomycin pretreatment. (c,d) Injection of IP3df into thapsigargin (Tg, 2 μM, 4 h)-treated cells did not induce any stimulation ofIClT. Cells incubated in vehicle alone (Ctr, 50 μM-free calcium L15) produce a largeIClTin response to IP3df. TheIClTcurrents were measured before and 20 min after IP3df injection. Data are means±s.e.m., the number of cells tested is indicated above each bar. Statistics: *P<0.05 and ***P<0.001; and NS, not significant. Figure 3: I ClT stimulation by IP 3 requires SERCA and active IP 3 R. ( a ) The injection of heparin (final concentration ~0.4 mg ml −1 ) inhibits the I CIT induced by IP 3 df injection. ( b ) The injection of IP 3 df still potentiates I ClT when the stores have been previously depleted with ionomycin (ion). The inset shows a bar chart summary of the time required to reach 25% maximal I ClT in control and ionomycin-pretreated cells. The data show a significantly more rapid rise ( P <0.001) with ionomycin pretreatment. ( c , d ) Injection of IP 3 df into thapsigargin (Tg, 2 μM, 4 h)-treated cells did not induce any stimulation of I ClT . Cells incubated in vehicle alone (Ctr, 50 μM-free calcium L15) produce a large I ClT in response to IP 3 df. The I ClT currents were measured before and 20 min after IP 3 df injection. Data are means±s.e.m., the number of cells tested is indicated above each bar. Statistics: * P <0.05 and *** P <0.001; and NS, not significant. Full size image To further test this model, we depleted Ca 2+ stores with ionomycin (20 s application) to activate SOCE, a treatment that does not activate I ClT significantly ( Fig. 3b ). Remarkably, under these conditions where SOCE is already activated, robust I ClT can be stimulated following injection of IP 3 df to gate open IP 3 Rs and allow Ca 2+ release from the ER ( Fig. 3b ). Consistently, the rate of rise of I ClT in response to IP 3 df injection was significantly faster when cells were pretreated with ionomycin ( Fig. 3b , inset). These experiments show that in the same cell, store depletion is not sufficient to efficiently activate CaCC, rather active IP 3 Rs are also required to allow Ca 2+ flowing through SOCE channels to be detected by CaCCs ( Fig. 3b ). These results support the model where Ca 2+ flowing through SOCE is taken up by SERCA into ER stores, and then released again through IP 3 Rs in close physical proximity of CaCCs, thus enhancing the efficiency of SOCE-mediated Ca 2+ influx in activating a primary downstream effector, the CaCCs. We therefore inhibited SERCA activity with thapsigargin resulting in store depletion, and then injected IP 3 df to activate IP 3 Rs ( Fig. 3c ). This experimental paradigm did not result in the activation of large I ClT ( Fig. 3c,d , Tg). In contrast, injection of IP 3 df in control-untreated cells displayed a normal large I ClT response ( Fig. 3c,d , Ctr). This shows that SERCA-mediated store refilling is required for efficient activation of CaCC following IP 3 generation and SOCE activation. Collectively, these results strongly argue that Ca 2+ ions flowing through SOCE channels transit through the ER lumen before reaching their target, the CaCCs. To test whether this functional coupling between SOCE, SERCA and IP 3 R is efficient at activating CaCC at the physiological resting membrane potential of the oocyte (~ −30 mV), we followed I Cl1 development following store depletion with IP 3 or ionomycin ( Supplementary Fig. 4 ). As with I ClT , I Cl1 preceded by a −30 mV voltage pulse activates only following IP 3 and not ionomycin treatment ( Supplementary Fig. 4 ). CaCC and SOCE clusters localize to distinct membrane domains The conclusions reached based on the functional data make specific predictions regarding the spatial distribution of the SOCE machinery, SERCA pumps, IP 3 Rs and CaCCs as downstream effectors. To investigate the spatial distribution of these proteins, we used YFP-tagged STIM1 to mark the STIM1-Orai1 SOCE clusters and cherry-tagged TMEM16A to visualize CaCCs. At rest, STIM1 localizes to the ER and CaCCs localize to the cell membrane ( Fig. 4a , Ctr). IP 3 -mediated store depletion results in the translocation of STIM1 to the cortical ER domain just below the cell membrane, where it co-localizes in clusters with Orai1 in a single focal plane as visualized in cells co-expressing STIM1 and Orai1 ( Supplementary Fig. 5B ) [45] , [47] . In contrast to Orai1, which localizes to the STIM1 clusters following store depletion, CaCCs remain diffusely distributed at the cell membrane, but are excluded from the STIM1 puncta ( Fig. 4a , IP 3 ). This is apparent in the orthogonal section across the z-stack of images and in the three-dimensional (3D) reconstruction through the cell membrane ( Fig. 4a , IP 3 ), and in the high magnification image in Fig. 4c (top panel), which shows the exclusion of the CaCCs from the SOCE puncta defined by STIM1. To quantify STIM1 and CaCC co-localization, we measured the Pearson’s co-localization coefficient after store depletion in cells expressing Ch-TMEM16A and YFP-STIM1, with the positive control for high co-localization provided by cells expressing Orai1 and STIM1 ( Fig. 4b ) [48] . The very low Pearson’s coefficient for TMEM16A/STIM1 as compared with the one obtained for STIM1/Orai1 after store depletion is consistent with the active exclusion of CaCCs from the STIM1-Orai1 puncta. Therefore, store depletion broadly defines two distinct domains at the cell membrane: the SOCE microdomain outlined by Orai1-STIM1 clusters and the membrane domain painted by CaCCs devoid of STIM1-Orai1 clusters. This shows that CaCCs are excluded from SOCE microdomain, which explains the need for active IP 3 Rs to allow for efficient transfer of Ca 2+ flowing through SOCE to activate CaCCs. 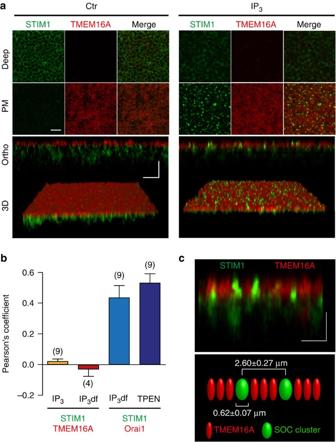Figure 4: Subcellular localization of TMEM16A, STIM1 and Orai1. (a) Cells expressing YFP-STIM1 and TMEM16A-mCherry were imaged by confocal microscopy. A z-stack of images was collected and reveals the typical reticular pattern and intracellular localization of YFP-STIM1 (Deep) as well as the expression of the CaCC (TMEM16A-mCh) at the plasma membrane (PM) before store depletion (Ctr). An orthogonal section across the z-stack of images and 3D reconstruction of the stack (below) show distinct localization of both proteins. After store depletion with IP3YFP-STIM1 can be found in dense clusters that translocate to the cortical ER within the PM focal plane. TMEM16A-mCh segregates away from STIM1 clusters and is distributed diffusely across the PM. Scale bars, 5 μm. (b) Pearson’s coefficient was used to evaluate and compare the co-localization of STIM1 with TMEM16A or Orai1 after store depletion with different agents (IP3, IP3df or TPEN). (c) Enlarged view of the STIM1 clusters and TMEM16A in an orthogonal section of the PM (upper panel). The lower panel shows a cartoon depicting the measured spatial parameters of the STIM1 clusters (see Methods section). The vertical scale bar represent 5 μm and the horizontal bar represents 1 μm. Figure 4: Subcellular localization of TMEM16A, STIM1 and Orai1. ( a ) Cells expressing YFP-STIM1 and TMEM16A-mCherry were imaged by confocal microscopy. A z-stack of images was collected and reveals the typical reticular pattern and intracellular localization of YFP-STIM1 (Deep) as well as the expression of the CaCC (TMEM16A-mCh) at the plasma membrane (PM) before store depletion (Ctr). An orthogonal section across the z-stack of images and 3D reconstruction of the stack (below) show distinct localization of both proteins. After store depletion with IP 3 YFP-STIM1 can be found in dense clusters that translocate to the cortical ER within the PM focal plane. TMEM16A-mCh segregates away from STIM1 clusters and is distributed diffusely across the PM. Scale bars, 5 μm. ( b ) Pearson’s coefficient was used to evaluate and compare the co-localization of STIM1 with TMEM16A or Orai1 after store depletion with different agents (IP 3 , IP 3 df or TPEN). ( c ) Enlarged view of the STIM1 clusters and TMEM16A in an orthogonal section of the PM (upper panel). The lower panel shows a cartoon depicting the measured spatial parameters of the STIM1 clusters (see Methods section). The vertical scale bar represent 5 μm and the horizontal bar represents 1 μm. Full size image To measure the size and distribution of these two distinct PM domains after store depletion, we calculated the average span of STIM-Orai puncta in the oocyte at 0.62+0.07 μm, and the average distance between these puncta, which defines the CaCC-positive domain, at 2.6+0.27 μm ( Fig. 4c ). Therefore, for Ca 2+ ions entering the cell through SOCE to fully activate CaCCs they would need to travel a minimum of ~1 μm. This distance is an underestimate and could be significantly larger given the microvilli rich structure of the oocyte cell membrane, because microvilli extend up to 3 μm. As is apparent in the case of ionomycin-dependent store depletion ( Fig. 1c,d ), Ca 2+ flowing through SOCE is inefficient at spanning this distance to effectively stimulate CaCC. This is likely due to Ca 2+ uptake in the SOCE microdomain by SERCA and the cytoplasmic Ca 2+ buffering. IP 3 R localizes to the cortical ER away from SOCE puncta Collectively, the functional and spatial distribution data argue for a model where Ca 2+ flowing through SOCE channels is first taken up into the stores by SERCA and then released by IP 3 Rs to activate CaCCs. Consistently with this conclusion when the distribution of IP 3 Rs is visualized in cell co-expressing STIM1, both proteins co-localize to the bulk ER at rest ( Fig. 5a , Ctr). Store depletion leads to the movement of STIM1 to SOCE puncta, whereas the IP 3 R maintains its diffuse ER-specific staining pattern ( Fig. 5a , TPEN). These observations are confirmed by Pearson coefficient analysis of STIM1 and IP3R co-localization ( Fig. 5a , Pearson's Coefficient). This shows that IP 3 Rs do not co-cluster with STIM1 in the SOCE puncta, but rather remain diffusely distributed within the ER. This is reminiscent of the separation observed between SOCE puncta and CaCC distribution at the PM ( Fig. 4 ). Therefore, the segregation of IP 3 R and CaCC away from SOCE puncta following store depletion enhances the efficiency of Ca 2+ release from the ER. Although this model is intuitively attractive, for IP 3 R in the ER to able to effectively deliver Ca 2+ to CaCC at the PM they would need to be close enough to the cell membrane. IP 3 Rs deep within the ER would not be expected to provide an effective conduit to deliver Ca 2+ flowing through SOCE channels to CaCCs. To test whether IP 3 Rs are close enough to the cell membrane following store depletion, we used STIM1 distribution as a ruler to define the cortical ER domain. STIM1 clusters localize within 10–20 nm of the cell membrane to allow direct physical coupling between STIM1 and Orai1 (refs 35 , 49 , 50 ). To estimate the population of IP 3 Rs that localizes to the cortical ER, we measured the intensity profile of IP 3 R and STIM1 across the z-stack of confocal images ( Fig. 5a,b ). Using the STIM1 peak as a threshold to define the cortical ER plane, we calculated the percentage of IP 3 R within the cortical ER from the integral of the IP 3 R intensity curve as shown in Fig. 5b . Before store depletion, STIM1 and IP 3 R have a similar intensity profile, showing that both proteins localize to the deep ER ( Fig. 5a,b ). Store depletion leads to the translocation of the STIM1 protein pool to the cortical ER (41.0±3.8%, n =7 being localized in planes above the peak, Fig. 5b ), with a concomitant movement of a subset of IP 3 R to the cortical ER focal plane ( Fig. 5b ). This analysis reveals that 17.9±3.5% ( n =7) of the IP 3 R population localizes to the cortical ER and as such are ideally positioned to activated CaCCs ( Fig. 5b ). A similar analysis of the distribution of STIM1 and Orai1 shows the more marked translocation of STIM1 after store depletion ( Fig. 5b ). 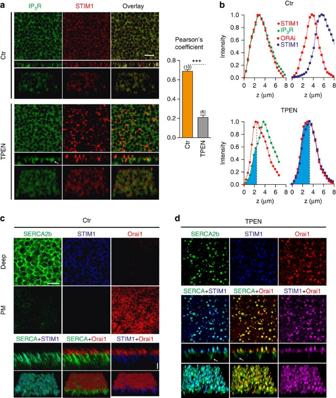Figure 5: Localization of IP3R, SERCA2b and STIM1. (a) Localization of GFP-IP3R and mCh-STIM1 before and after store depletion with TPEN. The upper panels are single focal planes, the middle panels are orthogonal sections along thezaxis and the lower panels are 3D reconstruction of the z-stacks. Pearson’s coefficient was used to evaluate co-localization of IP3R and STIM1 before and after store depletion. The two proteins localize at rest and store depletion significantly (P<0.001) decreases their co-localization. The horizontal scale bar represents 5 μm and the vertical bar 2.5 μm. (b) A subset of IP3R moves to the cortical ER following store depletion. The fluorescence intensity was plotted against the vertical position (z, orthogonal to the PM) to measure the translocation of proteins. Although STIM1 and IP3R are in identical focal planes at rest, Orai1 shows a distinct localization to the PM (upper panels, Ctr). After store depletion, while STIM1 and Orai1 localize to identical optical layers (TPEN, lower panel), only a fraction of IP3R translocates along with STIM1 to the cortical ER focal plane (left panel, highlighted in blue). This cortical localization of the IP3R following store depletion is apparent in the orthogonal section in panel A (arrow). (c) In resting conditions, GFP-SERCA2b and YFP-STIM1 co-localize in the ER compartment (deep) and display a reticular pattern. The horizontal scale bar represents 5 μm and the vertical bar represents 2.5 μm. (d) After store depletion, GFP-SERCA2b and YFP-STIM1 translocate to the PM optical plane where they co-localize with Orai1 and display a punctate pattern typical of cluster formation. Below each panel is an orthogonal and 3D reconstruction of the z-stack. The scale bars fromcapply. Statistics: ***P<0.001. Figure 5: Localization of IP 3 R, SERCA2b and STIM1. ( a ) Localization of GFP-IP 3 R and mCh-STIM1 before and after store depletion with TPEN. The upper panels are single focal planes, the middle panels are orthogonal sections along the z axis and the lower panels are 3D reconstruction of the z-stacks. Pearson’s coefficient was used to evaluate co-localization of IP 3 R and STIM1 before and after store depletion. The two proteins localize at rest and store depletion significantly ( P <0.001) decreases their co-localization. The horizontal scale bar represents 5 μm and the vertical bar 2.5 μm. ( b ) A subset of IP 3 R moves to the cortical ER following store depletion. The fluorescence intensity was plotted against the vertical position ( z , orthogonal to the PM) to measure the translocation of proteins. Although STIM1 and IP 3 R are in identical focal planes at rest, Orai1 shows a distinct localization to the PM (upper panels, Ctr). After store depletion, while STIM1 and Orai1 localize to identical optical layers (TPEN, lower panel), only a fraction of IP 3 R translocates along with STIM1 to the cortical ER focal plane (left panel, highlighted in blue). This cortical localization of the IP 3 R following store depletion is apparent in the orthogonal section in panel A (arrow). ( c ) In resting conditions, GFP-SERCA2b and YFP-STIM1 co-localize in the ER compartment (deep) and display a reticular pattern. The horizontal scale bar represents 5 μm and the vertical bar represents 2.5 μm. ( d ) After store depletion, GFP-SERCA2b and YFP-STIM1 translocate to the PM optical plane where they co-localize with Orai1 and display a punctate pattern typical of cluster formation. Below each panel is an orthogonal and 3D reconstruction of the z-stack. The scale bars from c apply. Statistics: *** P <0.001. Full size image The SERCA pump localizes to the SOCE puncta We next imaged the subcellular distribution of SERCA before and after store depletion in cells co-expressing STIM1 and Orai1 ( Fig. 5c,d ). At rest, SERCA co-localizes with STIM1 to the deep ER plane ( Fig. 5c , Deep), whereas Orai1 localizes to the PM plane. The distribution of SERCA, STIM1 and Orai1 at rest is visible in the orthogonal sections and 3D reconstructions ( Fig. 5c , lower panels). Store depletion results in the translocation of SERCA to the STIM1-Orai1 puncta at the PM–cortical ER focal plane ( Fig. 5d ). Although the majority of the STIM1 protein population moves to the cortical ER following store depletion, a significant proportion of the SERCA protein population remains in the deep ER as is apparent in the orthogonal sections in Fig. 5d (white arrows). Co-localization of SERCA with STIM1 and Orai1 in two-dimensional images, orthogonal sections and 3D reconstructions is apparent ( Fig. 5d ), showing that SERCA localizes to the SOCE microdomain consistent with previous findings [51] , [52] . Similar results were obtained when store were depleted with IP 3 ( Supplementary Fig. 6 ). The localization of SERCA to the SOCE clusters is consistent with the functional data showing that SERCA activity is essential for efficient activation of CaCC downstream of Ca 2+ influx through SOCE ( Fig. 3c ). Contribution of SOCE to membrane depolarization CaCC underlie the predominant current in the oocyte and contribute to setting the resting membrane potential, which ranges between −40 and −60 mV. P Cl /P K in the oocyte is estimated at 0.4 and E Cl at −24 mV consistent with a significant contribution of Cl − fluxes in setting the resting membrane potential [53] . To evaluate the physiological role of the interaction between SOCE, IP 3 R and CaCC, we recorded the effect of LPA on the oocyte membrane potential. Bath application of 1 μM LPA induced a biphasic depolarization of the cell consisting of a first transient phase followed by a second sustained plateau phase ( Fig. 6a ), which track with the Ca 2+ release from the ER and Ca 2+ influx from the extracellular space. Consistently, when the cells were treated with BTP-2 to inhibit SOCE, the first phase was unaffected, whereas the plateau phase was abolished ( Fig. 6a,b ). The first transient phase is therefore likely to be solely due to Ca 2+ release from stores, whereas the plateau phase matches the development of SOCE. Indeed when changes in membrane voltage are plotted concurrently with the development of I Cl1 and I ClT following LPA treatment, the first depolarization phase coincides with the activation of CaCC due to Ca 2+ release from stores ( I Cl1 ), whereas the sustained depolarization phase is due to SOCE-dependent activation of CaCC ( I ClT ) ( Fig. 6c ). Therefore, functional coupling between SOCE, SERCA and IP 3 R specifically activates CaCC and regulates the cell’s membrane potential, which is essential for cellular homeostasis and viability. 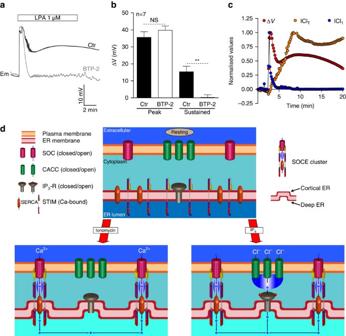Figure 6: SOCE-dependent CaCC activation regulates oocyte resting membrane potential. (a) The membrane potential (Em) of aXenopusoocyte was recorded using a single intracellular electrode. The application of LPA (1 μM) produces a biphasic depolarization. The second (sustained) phase of the depolarization can be inhibited by BTP-2 (10 μM), a SOCE inhibitor. (b) Bar chart summarizing the effects of BTP-2 on the peak and sustained component of the LPA-induced depolarization. (c) The graph illustrates the time course of the effect of LPA (1 μM) on the membrane potential (ΔV),ICl1andIClT. The values for the three parameters were normalized to the maximum and superimposed. The development ofIClTmatches the plateau phase of the membrane depolarization, whereas theICl1peak is synchronized with the fast membrane depolarization. (d) Model illustrating the functional coupling between SOCE, SERCA and IP3R following different modes of store depletion. Statistics: **P<0.01 and NS, not significant. Figure 6: SOCE-dependent CaCC activation regulates oocyte resting membrane potential. ( a ) The membrane potential (Em) of a Xenopus oocyte was recorded using a single intracellular electrode. The application of LPA (1 μM) produces a biphasic depolarization. The second (sustained) phase of the depolarization can be inhibited by BTP-2 (10 μM), a SOCE inhibitor. ( b ) Bar chart summarizing the effects of BTP-2 on the peak and sustained component of the LPA-induced depolarization. ( c ) The graph illustrates the time course of the effect of LPA (1 μM) on the membrane potential (Δ V ), I Cl1 and I ClT . The values for the three parameters were normalized to the maximum and superimposed. The development of I ClT matches the plateau phase of the membrane depolarization, whereas the I Cl1 peak is synchronized with the fast membrane depolarization. ( d ) Model illustrating the functional coupling between SOCE, SERCA and IP 3 R following different modes of store depletion. Statistics: ** P <0.01 and NS, not significant. Full size image The point-source introduction of Ca 2+ , into the cytosol through PM or ER Ca 2+ -permeable channels, results in a gradient of Ca 2+ with high Ca 2+ concentrations at the mouth of the channel that gradually decrease as Ca 2+ diffuses away and is captured by cytoplasmic buffers [6] . Such Ca 2+ microdomains are associated with SOCE and activate co-localized effectors, including volume-activated anion channel [54] , Ca 2+ -dependent adenylate cyclase [55] , [56] , [57] , phospholipase A2 (cPLA2), and 5-lipoxygenase to generate the pro-inflammatory leukotriene LTC4 in mast cells [5] , [58] . In fact adenylate cyclase-8 directly interacts with Orai1 [59] , explaining its exquisite activation through SOCE. However, other SOCE-dependent effectors such as CaCC and NFAT are efficiently activated by SOCE, yet localize away from the SOCE microdomain. Hence, Ca 2+ flowing in the SOCE microdomain is able to activate distal effectors without inducing a global Ca 2+ wave. This argues that cells have evolved mechanisms to allow for Ca 2+ signalling in the mid-range, between the microdomain and whole cell. However, the mechanisms regulating mid-range Ca 2+ signalling are unknown. Here we elucidate a mechanism that allow for SOCE-dependent Ca 2+ signalling in the mid-range. We show using the CaCC as Ca 2+ -dependent effectors of SOCE that Ca 2+ flowing through a cluster of SOCE channels in a spatially delimited domain is taken up effectively by the SERCA pump into the ER lumen, only to be released again through open IP 3 Rs that localize away from the SOCE cluster to activate CaCC (see model in Fig. 6d ). Therefore, the spatial extent of SOCE-dependent Ca 2+ influx is extended through functional coupling to IP 3 Rs. This mechanism allows cells to control the activation of Ca 2+ -dependent effectors that localize spatially away from the Ca 2+ signalling domain effectively and specifically without inducing a global Ca 2+ rise. Such a mechanism is likely to be at play downstream of SOCE in other cell types. For example, there is evidence in lymphocytes that NFAT translocation to the nucleus is more efficient following receptor stimulation when compared with store depletion alone [60] . Similarly, the activation of K Ca channels in human submandibular gland (HSG) cells by carbachol depends on both SOCE and receptor stimulation [15] . The functional coupling between SOCE-SERCA-IP 3 R to activate large CaCC is physiologically important as it regulates the membrane potential of the cell in response to agonist stimulation, which is critical for homeostasis and maintenance of basic functions such as nutrient and solute transport across the cell membrane. Furthermore, membrane potential deregulation has been associated with the induction of apoptosis in the oocyte [61] . Maintenance of the oocyte membrane potential is key for oocyte growth and development [21] . In summary, we describe the molecular mechanisms controlling mid-range Ca 2+ signalling. Uptake of Ca 2+ flowing through SOCE by SERCA into the ER and then Ca 2+ release through IP 3 Rs as illustrated in Fig. 6d allows for specific and efficient activation of CaCC that are excluded from the SOCE signalling microdomain. Such an arrangement is ideally suited for SOCE as it maintains low Ca 2+ concentration in the SOCE domain, thus slowing Ca 2+ -dependent inactivation of SOCE [62] , [63] and extending the duration of Ca 2+ influx. This prolonged SOCE-dependent Ca 2+ influx activates CaCCs in a spatially distinct domain through IP 3 R-dependent Ca 2+ release that is fuelled by Ca 2+ influx through SOCE. Therefore, store depletion leads to a spatial redistribution of membrane channels due to the formation of ER–PM junctions, which concentrate Orai1 while excluding CaCCs. This is accomplished while maintaining robust functional coupling between SOCE and CaCC, with the requirement for active IP 3 Rs to mediate this coupling. Physiologically, store depletion is coupled to the generation of IP 3 and as such activation of IP 3 R. However, in addition to its well-recognized role in the Ca 2+ release phase following agonist stimulation, we now show that the IP 3 R is also important in transmitting the SOCE signal to specific downstream effectors during the influx phase of Ca 2+ signalling. Molecular biology The constructs for mCh-STIM1, YFP-STIM1, Orai1-GFP, GFP-IP3R and TMEM16a-mCh have been previously described [45] , [47] , [64] . The GFP-tagged SERCA2b was a generous gift from James Lechleiter. All chemicals were obtained from Sigma except BTP-2 and IP 3 df (Calbiochem, Darmstadt, Germany), thapsigargin and ionomycin (Life Technologies, Grand Island, NY, USA). Expression in Xenopus oocytes Stage VI oocytes were harvested from wild-type adult Xenopus laevis females (Xenopus Express, France) using previously described procedures [26] . Briefly, frogs were anaesthetised using tricaine (5 g l −1 ) and the ovaries were surgically removed and cut open to allow easier enzymatic digestion. The oocytes were then defolliculated in collagenase type 1A (2 mg. ml −1 in Ca 2+ free Ringer) under gentle shaking then stored at 18 °C. Oocytes were kept in 0.5 × L15 (Sigma, St. Louis, MO, USA), for low Ca 2+ condition, free Ca 2+ was kept to 50 μM using EGTA. Typically, the cells were injected 24 h after harvesting and expression was allowed for at least 48 h. The injected RNA amounts were as follows: GFP-Orai1 2 ng, TMEM16A-mCh 8 ng mCh-STIM1 and YFP-STIM1 (10 ng), GFP-SERCA2b (20 ng) and GFP-IP3R (160 ng). Electrophysiology The ionic currents were recorded using standard two-electrode voltage-clamp recording technique. Recording electrodes were filled with 3 M KCl and coupled to a Geneclamp 500B controlled with pClamp 8.2 (Axon instruments). Intracellular Ca 2+ levels were monitored using Ca 2+ -activated chloride currents as sensors as previously described [40] . The cells were continuously superfused with saline during voltage-clamp experiments using a peristaltic pump. The standard extracellular saline contained (in mM) 96 NaCl, 2.5 KCl, 1.8 CaCl 2 , 2 MgCl 2 , 10 HEPES, pH 7.4. As outlined in Fig. 1a , endogenous CaCCs in the Xenopus oocyte allow the separation of Ca 2+ influx and Ca 2+ release using a triple-voltage jump protocol from a holding potential of −30 mV to a depolarization pulse at +40 mV followed by hyperpolarization to −140 mV and then depolarization again to +40 mV. The current during the first +40 mV depolarizing pulse is referred to as I Cl1 and reflects Ca 2+ release from intracellular stores (left traces and cartoon). The −140 mV hyperpolarization pulse increases the driving force for Ca 2+ entry into the cell and as such stimulates CaCC, a current referred to as I Cl2 ( Fig. 1a , right cartoon and trace). The third pulse is identical to the first one and measures the CaCC in response to Ca 2+ that entered the cell during the preceding hyperpolarization pulse, a current referred to as I ClT ( Fig. 1a , right trace). I ClT activates rapidly in response to the Ca 2+ that entered the cell during the −140 mV pulse and then decays gradually as Ca 2+ dissipates [40] . Imaging Confocal imaging of live cells was performed using a LSM710 (Zeiss, Germany) fitted with a Plan Apo × 63/1.4 oil immersion objective or a TCS SP5 (Leica, Germany) fitted with a × 63/1.4-0.6 oil immersion objective, z-stacks were taken in 0.5 μm sections using a 1 Airy unit pinhole aperture. The images were recorded with Zen2008 (Zeiss) or LAS AF 2.4.1 (Leica). For intracellular Ca 2+ imaging, the Zeiss LSM710 was fitted with a plan-Apochromat × 10/0.45 M27objective and a pinhole set to 1 Airy unit. The confocal scanner was synchronized with pClamp using a custom-made cable according to Zeiss specifications. The cells were injected before recording with 40 μM Oregon Green BAPTA-1. Images were analysed with ImageJ 1.46q (ref. 65 ). For cluster measurement purposes, thresholded images of the plane with maximum STIM1 clusters were used. All clusters were then measured using the ImageJ ‘Analyze particles’ function, the area of the detected particles was then measured. To remove non-specific particle detection, a cutoff value of twice the s.d. of the area of all detected particles was used. The distance between the selected clusters was then determined using the ‘nearest neighbor distance’ plugin. Statistics Values are given as means±s.e.m.. Statistical analysis was performed when required using either Student’s paired and unpaired t -test or analysis of variance followed by Newman–Keuls post hoc test. P values are indicated as follows: * P <0.05, ** P <0.01, *** P <0.001 and NS, not significant. Statistics were obtained using Prism 5.04 (GraphPad Software, La Jolla, CA, USA). Ethical approval Animals were handled according to Weill Cornell Medical College Institutional Animal Care and Use Committee (IACUC) approved procedures. How to cite this article: Courjaret, R. et al. Mid-range Ca 2+ signalling mediated by functional coupling between store-operated Ca 2+ entry and IP 3 -dependent Ca 2+ release. Nat. Commun. 5:3916 doi: 10.1038/ncomms4916 (2014).